Waving potential in graphene Nanoscale materials offer much promise in the pursuit of high-efficient energy conversion technology owing to their exceptional sensitivity to external stimulus. In particular, experiments have demonstrated that flowing water over carbon nanotubes can generate electric voltages. However, the reported flow-induced voltages are in wide discrepancy and the proposed mechanisms remain conflictive. Here we find that moving a liquid–gas boundary along a piece of graphene can induce a waving potential of up to 0.1 V. The potential is proportional to the moving velocity and the graphene length inserted into ionic solutions, but sharply decreases with increasing graphene layers and vanishes in other materials. This waving potential arises from charge transfer in graphene driven by a moving boundary of an electric double layer between graphene and ionic solutions. The results reveal a unique electrokinetic phenomenon and open prospects for functional sensors, such as tsunami monitors. According to the classical electrokinetic theory developed since 1808, a streaming potential can build up across a liquid flow through a narrow channel in proportion to the pressure difference applied across the channel [1] . Without the pressure gradient, no voltage can be detected in the flowing liquid. Nanoscale materials offer much promise in pursuing high-efficient energy conversion technology owing to their particular size and surface effects that introduce exceptional sensitivity to external stimulus [2] , [3] , [4] , [5] , [6] . Since 2001, a lot of attempts have been made to produce a voltage in carbon nanomaterials immersed in flowing liquid without the pressure gradient as required for the streaming potential [7] , [8] , [9] , [10] , [11] , [12] . However, the reported flow-induced voltages are in wide discrepancy and the proposed mechanisms remain conflictive [8] , [9] , [10] , [11] , [12] , [13] , [14] . The extensively studied two-dimensional graphene, a graphite monolayer with outstanding electronic and mechanical properties [15] , [16] , [17] , is now available in large area [18] , [19] to react to the liquid flow, but still obeys the classical electrokinetic theory that a monolayer or few-layer graphene sheet immersed in water flow or moving under water cannot produce detectable electricity as there is no pressure gradient [20] . In contrast to all the reported attempts to produce electricity from streaming over immersed solid surfaces, we find here that once a graphene sheet is being inserted into ionic solutions or a liquid–gas boundary is moving along the graphene sheet, a distinct voltage can be induced without pressure gradient. As the moving boundary vividly manifests as waving water surface along the graphene sheet, we term the voltage as waving potential. This waving potential is proportional to the inserting velocity and the sheet size. A 2 × 10 cm 2 -sized graphene sheet can produce voltage of up to 0.1 V with a short circuit current of 11 μA at a velocity of 1 m s −1 . The induced electricity can also be scalable simply by parallel and series connections, and is large enough to stimulate a sciatic nerve of a frog, inducing sharp contraction of the gastrocnemius muscle. Intensive experimental and theoretical analyses reveal that the electricity originates from the transfer of charges in graphene driven by the liquid–gas boundary. A capacitor-resistance model is proposed to describe the waving potential measured in our experiments. Waving potential in graphene Our monolayer graphene samples were grown by low-pressure chemical vapour deposition on copper foil [18] and identified by Raman characterization ( Supplementary Fig. 1 ) [21] . The experimental set-up is illustrated in Fig. 1a , where a monolayer graphene sample with size around 2 × 10 cm 2 was transferred onto a polyester terephthalate substrate [22] . Silver emulsion electrodes were patterned on the two ends of each graphene sample with robust ohmic contact. The electrodes and graphene edges were then protected by silicone to avoid exposing to the liquid. The graphene sample is periodically inserted into and pulled out from the surface of a 0.6-M NaCl aqueous solution (~3.5 wt% as in seawater) at a constant velocity v . Typical voltage responses measured between the two electrodes in a moving period are shown in Fig. 1b . During the inserting process, the produced voltage increases nearly linearly with the depth d of the graphene section inserted into the solution. At v =3.1 cm s −1 , the voltage increases to its peak of 3.3 mV just before the 10-cm-long sheet completely enters the solution. Once the graphene sheet is completely immersed in the solution, the voltage signal drops sharply to a resting voltage of about 0.2 mV within 0.2 s and keeps stable (inset of Fig. 1b ) regardless of whether the sheet keeps moving or not ( Supplementary Fig. 2 ). Once the top of the sample turns to rise out of the solution surface, the voltage signal switches swiftly to its inverse peak of −3.3 mV and then gradually decreases in amplitude with decreasing depth d , showing a mirror behaviour to the insertion-induced signal. The positive and negative peak voltages will repeat alternately to form a series of regular electric signals by continuously moving the sample across the liquid–air boundary. 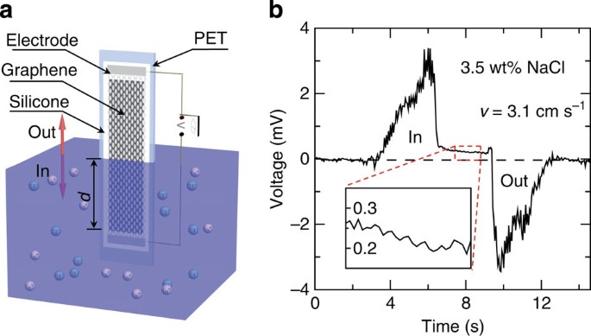Figure 1: Waving potential in graphene moving across the surface of seawater. (a) Schematic illustration of the experimental set-up: moving the graphene sample on a polyester terephthalate substrate vertically across the water surface within a container. All the edges of the graphene sheet and silver emulsion electrodes are protected with silicone. (b) Typical voltage signals produced as a sample is inserted and pulled out of 0.6 M NaCl solution (~3.5 wt%) at a velocityv=3.1 cm s−1. Figure 1: Waving potential in graphene moving across the surface of seawater. ( a ) Schematic illustration of the experimental set-up: moving the graphene sample on a polyester terephthalate substrate vertically across the water surface within a container. All the edges of the graphene sheet and silver emulsion electrodes are protected with silicone. ( b ) Typical voltage signals produced as a sample is inserted and pulled out of 0.6 M NaCl solution (~3.5 wt%) at a velocity v =3.1 cm s −1 . Full size image Mechanism analysis To our knowledge, this waving potential cannot be explained by any previously proposed mechanisms, such as phonon drag [10] , asymmetric fluctuating [7] or electronic friction [12] , because all the mechanisms are common in that the induced voltage should be observed with the sample moving completely under the water and without liquid–gas boundary being required, while in our experiments there is no measurable voltage under these conditions. Diffusio-osmosis effects [23] , arising from salt gradients, which may be introduced in our case by the water evaporation, are also excluded, since we did not find noticeable dependence of the induced voltage signal on the relative humidity ranging from 5 to 95% ( Supplementary Fig. 3 ). To understand the underlying physics, we first carry out first-principle calculations on the interaction of graphene with hydrated Na + and Cl − . The calculated adsorption energy is positive for Na + and negative for Cl − , indicating that graphene prefers to stick Na + (supported by the ab initio molecular dynamics simulations, Supplementary Fig. 4 ). In this way, an electric double layer (EDL) consisting of the firmly adsorbed Na + layer and attracted Cl − layer (known as diffuse layer) should form at the graphene–solution interface when reaching equilibrium. Moreover, an analysis of charge transfer shows that the graphene becomes hole doped by the EDL; the doping is even heavier when only a Na + layer adsorbs on graphene ( Fig. 2a , Supplementary Fig. 5 ). The EDL-enhanced hole doping is confirmed by our Hall measurements, showing that the hole concentration of graphene increases from 2.9 × 10 12 cm −2 in deionized water to 3.7 × 10 12 cm −2 in 1 mM NaCl ( Fig. 2a , right bottom). 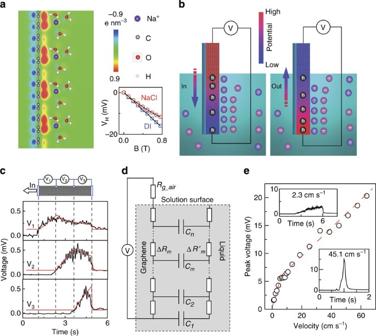Figure 2: Mechanism for the waving potential in a graphene sheet. (a) Charge redistribution of graphene upon adsorption of hydrated Na+(red for regions with charge accumulation and blue for charge depletion). Right bottom inset: Hall voltages as functions of magnetic field for graphene immersed in deionized water and 1 mM NaCl. (b) Schematic EDL and its boundaries by ion adsorption (left) and desorption (right) on the surface of graphene during the insertion and pulling out processes, respectively. Induced potential difference and hole concentration gradient in the graphene sheet are also illustrated. (c) Detected voltage signals of three subsections in graphene sample with four equally spaced electrodes (top inset). The dashed lines mark when the solution surface rises to the corresponding position of the sample in the top inset. The solid red lines are modelling results (Supplementary Note 2). (d) Equivalent circuit for the waving potential. (e) Peak voltage as a function of inserting velocityvof graphene into 0.6 M NaCl solution. The insets zoom in the signals atv=2.25 and 45.1 cm s−1. Figure 2: Mechanism for the waving potential in a graphene sheet. ( a ) Charge redistribution of graphene upon adsorption of hydrated Na + (red for regions with charge accumulation and blue for charge depletion). Right bottom inset: Hall voltages as functions of magnetic field for graphene immersed in deionized water and 1 mM NaCl. ( b ) Schematic EDL and its boundaries by ion adsorption (left) and desorption (right) on the surface of graphene during the insertion and pulling out processes, respectively. Induced potential difference and hole concentration gradient in the graphene sheet are also illustrated. ( c ) Detected voltage signals of three subsections in graphene sample with four equally spaced electrodes (top inset). The dashed lines mark when the solution surface rises to the corresponding position of the sample in the top inset. The solid red lines are modelling results ( Supplementary Note 2 ). ( d ) Equivalent circuit for the waving potential. ( e ) Peak voltage as a function of inserting velocity v of graphene into 0.6 M NaCl solution. The insets zoom in the signals at v =2.25 and 45.1 cm s −1 . Full size image During insertion of the graphene sheet into the solution, an EDL boundary will form near the gas–liquid interface on the graphene. The moving boundary of EDL determines that the adsorbed Na + ions nearby should be more abundant than Cl − ions, as the Cl − ions are relatively retarded in migration to form the diffuse layer (see Fig. 2b ). In this way, the net charge of Na + layer near the EDL boundary cannot be screened immediately by Cl − ions and therefore draws more electrons from graphene than do in the equilibrium EDL, thus raising local hole concentration and electric potential. The higher local potential drives a hole current from the boundary to the graphene section deeper in solution, where the hole concentration is lower as the EDL is closer to equilibrium ( Fig. 2b , left). Similarly, pulling out the graphene sheet drives the EDL boundary to move downwards and reverses the hole current ( Fig. 2b , right). To test this scenario, we measured the voltage distribution in the graphene sheet by vertically patterning four equally spaced electrodes and detecting the induced voltage in each subsection between two neighbouring electrodes (insert in Fig. 2c ). As the sheet is inserting into the solution, the voltage can be detected exclusively in the graphene section(s) beneath the solution surface ( Fig. 2c ). This means that the hole redistribution caused by the moving EDL boundary occurs only in the immersed graphene section. The voltage in each subsection increases as it is being inserted into the solution and peaks when the whole subsection is just immersed; then, it decays gradually as the boundary moves onto the next subsection in sequence. However, once the whole graphene sheet is completely immersed in the solution, the moving boundary disappears and the voltages in all the subsections drop abruptly to a resting voltage. The total voltage by summing up all the subsection voltages is close to the signal shown in Fig. 1b , with a peak voltage of 1.4 mV. By taking the immersed graphene sheet with adsorbed Na + as a positive plate and the Cl − diffusion layer as the negative plate, the EDL with moving boundary can be simplified as a series of equally spaced capacitors ( C 1 ~ C n ) connected in parallel, with equivalent series-connected resistances of Δ R 1 ~Δ R n for the immersed graphene section serving as the positive plate and Δ R 1 ′~Δ R n ′ for the solution serving as the negative plate, assuming the length of EDL is equally divided into n sections with equal density of Na + ions, as shown by the equivalent circuit in Fig. 2d . According to above discussion, when inserting graphene into solution, the capacitor C n at the moving EDL boundary will be more charged with higher potential than the rest capacitors C 1 ~ C n -1 lower in the solution. Thus, C n will discharge its charges equally to C 1 ~ C n -1 with a local current of I = q 0 Wv , where q 0 is the discharging charge per unit area of C n and W the width of the graphene sheet. The average current through each resistance should be ( Supplementary Note 1 ). Then, the voltage V detected in the graphene sheet can be expressed as where, x is the vertical distance from Δ R m of the graphene sheet to the liquid surface and R sq is the square resistance of graphene. Given an inserting velocity v , equation (1) shows a linear dependence of the induced voltage on the inserted depth d , in good agreement with the experimental results in Fig. 1b . This model is further confirmed by its excellent description of the dependence of measured voltage in each of the subsections on the inserted depth ( Fig. 2c , solid red lines; Supplementary Note 2 ). When the whole sheet is inserted into the solution, d reaches its maximum L , the length of graphene sheet clamped between two end electrodes, resulting in a peak voltage as . V peak hence increases with inserting velocity, which agrees again with the experimental results shown in Fig. 2e . In the low range of v ≤5.5 cm s −1 , V peak is in perfect proportion to v with a slope of 0.88 mV cm −1 s. However, for v >5.5 cm s −1 , the slope decreases to 0.25 mV cm −1 s, rendering a piece-linear behaviour, as fitted by the dashed lines in Fig. 2a . We attributed this lower slope at higher inserting velocity to the influence of the intrinsic wetting velocity of the graphene sample. Waving potential in a variety of ionic solutions The above results are common for other ionic solutions. The calculated adsorption energies of various hydrated cations/anions on graphene are shown in Fig. 3a , together with the bare cations/anions for comparison. Similar to the NaCl solution, all hydrated cations have positive adsorption energies over 2 eV while hydrated anions remain repulsive to graphene, enabling them to form essentially the same EDL. 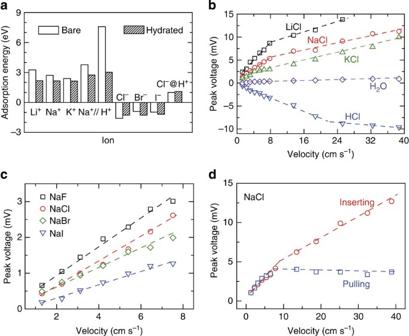Figure 3: Ion- and velocity-dependent waving potential. (a) Calculated adsorption energies of different ions on one side of monolayer graphene. Na+// is the value for a Na+adsorbed on a bilayer graphene. (b) Induced peak voltages as functions of velocity of graphene inserting into LiCl, NaCl, KCl and HCl solutions with the same concentration of 0.6 M as well as into deionized water. (c) Peak voltages as functions of velocity of graphene insertion into a series of halide sodium solutions. (d) The magnitudes of positive- and negative-peak voltages as functions of moving velocity of graphene across the surface of 0.6 M NaCl solution. Thus, the waving potential in graphene shows the same order and polarity in salt solutions of LiCl, KCl, NaF, NaBr and NaI at the same concentration of 0.6 M ( Fig 3b,c ). It is interesting that the waving potential is stronger in solutions with smaller cations or anions. Possible reasons should include the difference in ion adsorption density, hydration size and ability to response to the moving boundary. It is found that the induced voltage increases by ~70% as the NaCl solution being diluted from 0.6 to 0.01 M. However, the influence of ionic concentration becomes weak for concentration in the range from 0.2 to 1.8 M ( Supplementary Fig. 6 ). In deionized water nearly rid of ions, the waving potential is over one order lower. Figure 3: Ion- and velocity-dependent waving potential. ( a ) Calculated adsorption energies of different ions on one side of monolayer graphene. Na + // is the value for a Na + adsorbed on a bilayer graphene. ( b ) Induced peak voltages as functions of velocity of graphene inserting into LiCl, NaCl, KCl and HCl solutions with the same concentration of 0.6 M as well as into deionized water. ( c ) Peak voltages as functions of velocity of graphene insertion into a series of halide sodium solutions. ( d ) The magnitudes of positive- and negative-peak voltages as functions of moving velocity of graphene across the surface of 0.6 M NaCl solution. Full size image A special point is that the waving potential in the HCl solution is inversed in sign from that in salt solutions. Our first-principle calculations predict that H 3 O + cations in the HCl can be adsorbed on graphene much more strongly [20] , as confirmed by the electrochemical analyses ( Supplementary Fig. 7 ) and Raman characterization ( Supplementary Fig. 8 ). Therefore, the graphene sample in HCl solution will be highly p doped owing to the strongly adsorbed H 3 O + group. This positively charged H 3 O + -graphene sheet becomes attractive to Cl − with estimated adsorption energy over 1 eV, comparable to that of Na + on graphene ( Fig. 3a ). Then, the same model can be applied to the dynamic adsorption of Cl − onto the H 3 O + -graphene sheet, leading to a waving potential inverse in sign to that in salt solutions. This reversed voltage is even maintained in the first cycle of moving the HCl-wetted graphene sheet across the surface of NaCl solution, and then it recovers to the typical signal observed in NaCl solution in the repeated wetting cycles owing to the desorption of H 3 O + ( Supplementary Fig. 9 ), confirming the proposed mechanism. When pulling the graphene sheet out of the NaCl solution, desorption of Na + reduces the local potential of graphene sheet at the solution surface ( Fig. 2b ). Thus, holes flow upwards from the immersed section to that near the solution surface, causing a current and voltage reverse to the inserting signal. The dependence of V peak on the pulling velocity is presented and compared with the inserting curve in Fig. 3d . The pulling-induced V peak also linearly increases in magnitude with v below a critical value, but stays almost constant when the velocity is larger than the critical dewetting speed that now dominates the process of separating water from the graphene. The time for complete dewetting is estimated to be 0.5~1 s, although graphene on the polyester terephthalate substrate keeps hydrophobic, see Supplementary Fig. 10 . Typically, the turning point in the slope of dV peak / dv is almost the same for the inserting and pulling processes ( Fig. 3d ), but it varies with different ionic solutions ( Fig. 3b ), possibly attributed to their different wetting behaviours on graphene. Demonstration of using and enhancing the waving potential The proposed model also informs that the induced electricity can be effectively enhanced by increasing v . At v ~1 m s −1 , a typical graphene sample with a size of 2 × 10 cm 2 can generate an open circuit voltage of 0.1 V ( Supplementary Fig. 11 ), with a short circuit current up to 11 μA. Nevertheless, the negative V peak is far lower than the positive V peak at such a high v , as limited by the dewetting speed as in Fig. 3d . Using the electric output of the graphene sheet, we have successfully stimulated a sciatic nerve of a frog. In the left insert of Fig. 4a , two terminal electrodes of the graphene sheet were connected to the white corded sciatic nerve. The thigh bone was fixed, and the gastrocnemius muscle was connected to a force sensor firmly by a fine thread. Under the input electric pulse generated by inserting the graphene sheet into 0.1 M NaCl solution at ~1 m s −1 , a significant contraction of the gastrocnemius muscle was stimulated, as highlighted by the middle insert in Fig. 4a , producing a tensile force of about 3.8 g as recorded in Fig. 4a . 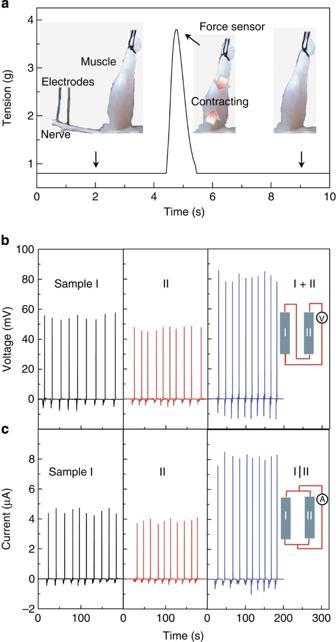Figure 4: Device demo of the waving potential and the scalability. (a) Contraction force detected by a force sensor connected to gastrocnemius muscle of a fog. Insets show contraction of the muscle by stimulating its sciatic nerve using the waving potential of a graphene sheet being inserted into 0.6 M NaCl solution at ~1 m s−1: original state (left), contracting state (middle) and restored state to original (right). (b) Series connection of graphene samples I and II (2 × 10 cm2, ~11 kΩ) across the surface of 0.6 M NaCl solution atv=55 cm s−1can amplify the produced voltage (I+II). (c) Parallel connection of the two samples can scale up the current (I|II). Insets illustrate how the samples are connected together for measurements. Figure 4: Device demo of the waving potential and the scalability. ( a ) Contraction force detected by a force sensor connected to gastrocnemius muscle of a fog. Insets show contraction of the muscle by stimulating its sciatic nerve using the waving potential of a graphene sheet being inserted into 0.6 M NaCl solution at ~1 m s −1 : original state (left), contracting state (middle) and restored state to original (right). ( b ) Series connection of graphene samples I and II (2 × 10 cm 2 , ~11 kΩ) across the surface of 0.6 M NaCl solution at v =55 cm s −1 can amplify the produced voltage (I+II). ( c ) Parallel connection of the two samples can scale up the current (I|II). Insets illustrate how the samples are connected together for measurements. Full size image Of practical importance is that the induced voltage and current at lower v are scalable simply through series and parallel connections of multiple graphene sheets as shown in Figs 4b-4c , respectively. This scalability can be understood straightforwardly from equation (1), which shows scalable V peak with increasing sheet length. Series connection of multiple graphene sheets increases the equivalent sheet length, while parallel connection increases the equivalent sheet width. When inserting a bi- or tri-layer graphene sheet of the same size into the NaCl solution, the induced voltage becomes one order lower than that in monolayer graphene ( Supplementary Fig. 12 ), mainly owing to significant reduction in the square resistance of these multilayered graphene samples. When inserting a thin sheet of other materials, such as graphite film, gold nanofilm, copper microfoil and doped silicon thin film into the ionic solutions, the induced voltages are measured to be at least two orders lower ( Supplementary Fig. 13 ). These results feature a unique behaviour of graphene in producing the waving potential from a few to hundred millivolts. Of more interest is that decreasing environment temperature from 45 to 6 °C leads to monotonic enhancement in the induced waving potential in graphene by about 40% ( Supplementary Fig. 14 ), possibly because of the suppressed thermal fluctuation of the EDL. As has been argued in previous reports [20] , whether the graphene samples used in this work could produce potential without the moving EDL boundary needs to be checked. Our careful experiments confirm again no detectable voltage even at the order of microvolt when the graphene samples are completely immersed in the solution with either symmetric or asymmetric electrodes being used, if only the electrodes are insulated from contacting with the solution ( Supplementary Fig. 15 ). In summary, we have demonstrated by systematic experimental investigations that a potential can be produced in a monolayer graphene sheet waving across air–solution interfaces. Different from the streaming potential built in flowing ionic solutions through narrow channels under high pressure gradient, the waving potential reported here is built in the graphene sheet by a moving liquid–gas boundary along it, in proportion to the moving velocity and the sheet size. Therefore, it can be scalable simply by series or parallel connection of multiple graphene sheets. This novel electrokinetic phenomenon based on an EDL with moving boundary can be used to design self-powered sensors and monitors, such as remote devices in the waving ocean. Experiment The graphene samples were grown using low-pressure chemical vapour deposition on 25 μm thick copper foil (Alfa Aesar, item number 13382) [18] . The as-grown graphene samples were then transferred onto a polyester terephthalate substrate according to the method developed by Ruoff and co-workers [22] . The induced voltage signal in graphene samples was recorded by a KEITHLEY 2010 multimeter, and the corresponding current was measured by a KEITHLEY 2400 multimeter. These meters were implemented by controlling software in a computer, and the sampling rate of our instruments is 20 s −1 . Theory The calculations were performed within the density functional theory framework as put into practice in the Vienna Ab-initio Simulation Package code [24] , [25] . We used the projector-augmented wave method [26] for the core region and the generalized gradient approximation of the Perdew-Burke-Ernzerhof functional for the exchange-correlation potential, with the energy cutoff set to 530 eV. The graphene sheet was modelled with a 5 × 5 supercell. The ions were simulated by adjusting the charge neutrality level with a uniform jellium countercharge and considering dipole correction to the total energy. The hydrated effect was simulated using up to six water molecules to surround the ions. The systems were fully relaxed without any constraint. How to cite this article: Yin, J. et al. Waving potential in graphene. Nat. Commun. 5:3582 doi: 10.1038/ncomms4582 (2014).